Synthesis ofmeta-carbonyl phenols and anilines Phenols and anilines are of extreme importance for medicinal chemistry and material science. The development of efficient approaches to prepare both compounds has thus long been a vital research topic. The utility of phenols and anilines directly reflects the identity and pattern of substituents on the benzenoid ring. Electrophilic substitutions remain among the most powerful synthetic methods to substituted phenols and anilines, yet in principle achieving ortho - and para -substituted products. Therefore, the selective preparation of meta -substituted phenols and anilines is the most significant challenge. We herein report an efficient copper-catalyzed dehydrogenation strategy to exclusively synthesize meta -carbonyl phenols and anilines from carbonyl substituted cyclohexanes. Mechanistic studies indicate that this transformation undergoes a copper-catalyzed dehydrogenation/allylic hydroxylation or amination/oxidative dehydrogenation/aromatization cascade process. Phenols and anilines are core structures of pharmaceuticals, agrochemicals, polymers, dyestuffs and natural products [1] , [2] , [3] , [4] . The development of efficient approaches to preparing both compounds has thus long been a vital research topic. Current strategies to synthesize phenols mainly include: (1) direct oxidation of the C(sp 2 )−H bond [5] , [6] , [7] , [8] , [9] , [10] (Fig. 1a(i) ); (2) transition metals-assisted conversion of the C(sp 2 )−X bond [11] , [12] , [13] , [14] , [15] (Fig. 1a(ii) ); (3) oxidation of the C(sp 2 )−M bond [16] , [17] (Fig. 1a(iii) ). In 2011, Stahl et al. reported an elegant palladium-catalyzed aerobic dehydrogenation of substituted cyclohexanones to phenols [18] (Fig. 1a(iv) ); and recently Tu et al. developed a dehydrogenation-coupling protocol to synthesize ortho -substituted phenols via cyclohexanones from cyclohexanols [19] . Compared to phenols, the synthesis of anilines from a corresponding C(sp 2 )–H bond involves multistep sequences and/or harsh conditions. For instance, it was first converted into nitro, nitroso, azo, azide, imine, or amide/imide/sulfonamide, followed by one or more additional steps to arrive at an amine [20] (Fig. 1a(v) ). Thanks to the development of metal-promoted reactions for over a century, three great name reactions, namely Ullmann−Goldberg reaction [21] , [22] (Fig. 1a(vi) ), Buchwald−Hartwig reaction [23] , [24] , [25] (Fig. 1a(vii) ), and Chan−Lam reaction [26] , [27] , [28] (Fig. 1a(viii) ) have been sequentially explored for the formation of C(sp 2 )-N bonds. These reactions have become fundamental tools for the preparation of anilines in numerous areas of basic and applied research [29] , [30] . However, all of these procedures are restricted by the need for a prefunctionalized arene, such as aryl halides, aryl pseudohalides, aryl organoborons, etc. Here, we present an alternative approach for the synthesis of phenols and anilines from carbonyl-substituted cyclohexanes (Fig. 1a(ix) ). Fig. 1: Synthesis of meta -carbonyl phenols and anilines. a Synthesis of phenols and anilines. b Recent work. c Proposed reaction process. Full size image The utility of phenols and anilines directly reflects the identity and pattern of substituents on the benzenoid ring. Therefore, the introduction of chemical functional groups on the specific site of their benzenoid ring represents a key point. Electrophilic aromatic substitutions (S E Ar) are classical chemical reactions that remain among the most powerful synthetic methods to substituted phenols and anilines, in principle achieving ortho - and para -substituted products due to the strong electron-donating nature and directing effects of the hydroxyl group and amino group. While the innate site selectivity limits the production of meta -substituted phenols and anilines, it yet has been inspiring extensive efforts of synthetic chemists to break through the limitation. In the past decades, the transition metal–catalyzed C–H activation strategy has provided a significant access to this challenge; and these methods mainly relied on: ruthenium-catalyzed σ-bond activation, remote directing template introduction, noncovalent interaction (e.g., hydrogen-bonding and ion-pair interaction), norbornene and a carboxylic acid group traceless assistance, steric hindrance effects, etc. [31] . Despite their high efficiency for meta -C(sp 2 )–H functionalization of phenols and anilines, these approaches required numerous functional group additions or manipulations in order to furnish the desired product. Furthermore, all of these methods inevitably generated a certain ration of ortho - and para -isomers; ortho -, meta -, and para -isomers always possess similar polarity and physical properties, thus their separation is always difficult. And it is known that the purification of the product is a key issue in industrial manufacturing. Herein, we disclose a specific synthesis of meta -substituted phenols and anilines by a copper-catalyzed dehydrogenation-allylic oxidation or amination-dehydrogenative aromatization sequence without ortho - and para -isomers detected. In the protocol, the Cu-catalyst plays crucial roles not only in promoting the dehydrogenation/allylic hydroxylation/oxidative dehydrogenation/aromatization cascade processes, but also in controlling the chemo- and regioselectivities. Inspired by recent work on the synthesis of 1,4-enediones from saturated ketones [32] (Fig. 1b ) and related literature [33] , [34] , we hypothesized that a similar process might proceed when cyclohexyl took the place of the alkyl chains moiety of ketones, and if that was followed by further dehydrogenation and aromatization, meta -functionalized phenols would be obtained (Fig. 1c ). However, the cascade transformation is challenging in view of the previous report where the cyclic ketone substrate generated a fully dehydrogenative aromatized product under dehydrogenation conditions [35] . 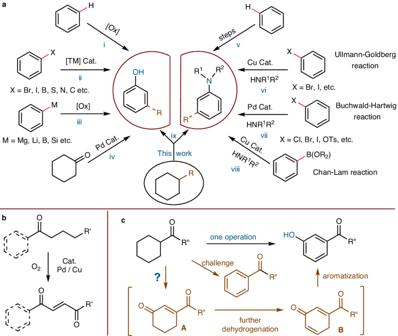Fig. 1: Synthesis ofmeta-carbonyl phenols and anilines. aSynthesis of phenols and anilines.bRecent work.cProposed reaction process. Reaction development The initial investigation began with cyclohexyl(phenyl)methanone 1a as the model substrate in the presence of Pd(OAc) 2 (10 mol%), Cu(OAc) 2 (10 mol%) and trifluoroacetic acid (TFA, 10.0 equiv) in DMSO (0.25 M) at 90 o C under O 2 for 60 h (Table 1 ). As expected, the desired meta -carbonyl product 2a was obtained, albeit in a low yield of 6% (entry 1). We also predictably detected the formation of small amounts of completely dehydrogenative aromatized byproduct 5 , as well as para -functionalized product 6 in the reaction, which motivated us to turn our attention to improving the yield and chemo- and regioselectivities of the reaction. Then with Pd(OAc) 2 as the catalyst, the other copper salts were investigated. The desired product 2a was obtained in 16% yield, with almost negligible product 6 , when CuI was employed as the co-catalyst (entry 2). Replacement of CuI with other copper salts led to inferior results (entry 3). In light of these results, we assumed that the CuI catalyst might have a vital impact on the yield and selectivity of the reaction. Indeed, the targeted 2a was delivered in 41% yield in the presence of CuI without Pd catalyst, whereas omission of CuI only led to a small quantity of 2a , indicating that CuI was key catalyst to convert 1a into the corresponding meta -carbonyl product 2a (entries 4 and 5). Further, we investigated other metal (e.g., Ni, Fe, Co and Ag) salts as co-catalysts or oxidants to improve the yield of 2a (entries 6–10). The experiments revealed that most Ag salts could contribute to high yields, while other metal salts proved ineffective (entries 9 and 10), and AgOAc emerged as the most productive co-catalyst for the reaction, providing the targeted product 2a in 53% yield (entry 9). Note that the ratio of AgOAc to CuI was crucial for the reaction. It was found that a larger amount of AgOAc inhibited the reactivity, while AgOAc (9 mol%) provided 2a in 64% yield (entry 11). Furthermore, when H 2 O (50 μL, 11.1 equiv) as an additive was introduced into the reaction system, 3 and 4 were completely consumed, improving the yield to 76% (entry 12). This result implies that water additive accelerates the transformation of 3 and 4 into 2a and also suggests that 3 and 4 were likely reaction intermediates to produce 2a (Supplementary Information Section 5.4 ). Moreover, the use of 18 O-labeled water provided the desired product with 18 O incorporation, showing the hydroxyl introduced into the products did come from the water [36] (Supplementary Fig. 5 ). A series of control experiments revealed that all the parameters in the reaction system were essential for the reaction to proceed; omission of either CuI or TFA resulted in no reaction (entries 11, 13–16). Alternatively, the reaction could also proceed in excellent yield under silver-free conditions, when using tert -butyl hydroperoxide (TBHP) instead of AgOAc and O 2 (entry 17). Table 1 Optimization of reaction conditions a Full size table Substrate scope Under the optimized conditions, we subsequently studied the substrate scope of the reaction (Fig. 2a ). A wide range of aryl ketones bearing various substituent groups all performed well, affording the corresponding meta -carbonyl phenols in good to excellent yields ( 2a – 2r ). Substrates containing electron-donating ( 2b, 2c, 2h – 2j , and 2n - 2q ) and electron-withdrawing ( 2d – 2g, 2k – 2m , and 2r ) groups on the aromatic ring were all well compatible, delivering the corresponding products in 51 to 88% yield. Halogens such as fluorine ( 2d, 2k , and 2r ), chlorine ( 2e and 2l ), bromine ( 2f ) and iodine ( 2g ) were tolerated, giving the desired products in good yields. Di- and tri-substituted aromatic substrates also reacted smoothly under the standard reaction conditions to generate the corresponding products ( 2s - 2v ). In addition, other aromatic or heterocyclic substrates such as naphthyl, furyl, thienyl, and benzothienyl were also applicable, as exemplified with products 2y, 2z, 2aa , and 2ab , furnished in up to 81% yield ( 2y – 2ab ). The structure of 2k was confirmed by single-crystal X-ray diffraction (Supplementary Information Section 6 ). The scalability of this reaction was investigated by a 5.5 mmol scale reaction of cyclohexyl(phenyl)methanone 1a , in which the desired product 2a could be obtained in 65% isolated yield (Supplementary Information Section 3.3 ). Fig. 2: Substrate scope for synthesis of meta -carbonyl phenols. a Substrate scope of aryl ketones. b Substrate scope of conjugated enones. c Substrate scope of aliphatic ketones and aldehydes. Reaction conditions: substrate (0.25 mmol), CuI (10 mol%), AgOAc (9 mol%), and TFA (10.0 equiv) in DMSO (1 mL), H 2 O (50 μL) under O 2 at 90 o C for 60 h. Isolated yields are reported. a Reaction conducted with 1a (5.5 mmol). b AgOAc (9.5 mol%) was used. c 48 h. d 100 o C. e No addition of H 2 O. f Pd(OAc) 2 (15 mol%) was used instead of AgOAc. Full size image Notably, conjugated enones 7 were also suitable for this transformation, producing bioactive chalcone derivatives in high yields ( 8a - 8l ), which further extends the diversity of this reaction (Fig. 2b ). Functional groups such as methyl ( 8b, 8e , and 8g ), methoxy ( 8h ), methylthio ( 8i ), alkynyl ( 8d ), and chlorine ( 8c and 8f ) were well tolerated, giving the meta -carbonyl phenols in 53–83% yield. Additionally, heterocyclic substrates were also well behaved with high efficiency ( 8k and 8l ). Interestingly, in addition to conjugated enones, conjugated dienones were also amenable to the standard conditions, generating products 8m to 8r in excellent yields regardless of their electronic properties. The structure of 8a was confirmed by single-crystal X-ray diffraction (Supplementary Information Section 6 ). To further expand the scope of this reaction, we next investigated other aliphatic ketones and aldehydes 9 (Fig. 2c ). By slightly tuning the reaction conditions, norfenefrine and etilefrine precursor 10a could be successfully synthesized. The cyclopropane ring, a highly reactive group, remained intact in the reaction, demonstrating the reaction conditions were mild. It should be mentioned that the product from ketone with α -methylene C−H bonds provided benzyl-oxygenated meta -carbonyl phenol 10c . The aliphatic ketone with α -quaternary center was amenable to the oxidative conditions, giving the expected product 10d . Of note, cyclic aldehydes, which are sensitive to oxidizing conditions, were also compatible with this transformation and furnished their corresponding products in high yields ( 10e and 10f ). It is well-known that ketone and aldehyde could be converted into various other groups, such as alkane, alkene, alcohol and acid, thus various meta -substituted phenols could be synthesized by this approach (Supplementary Information Section 5.7 ). Buoyed by the success in the synthesis of meta -carbonyl phenols, we turned our focus on the synthesis of meta -carbonyl anilines. As mentioned above, the hydroxyl group of meta -carbonyl phenols came from water in this reaction system. It is reasonable that, instead of water, the introduction of amine into the reaction system would produce meta -carbonyl anilines. Thus, we investigated the reaction between cyclohexyl(phenyl)methanone 1a and aniline 11a under the standard reaction conditions. As anticipated, the expected meta -carbonyl aniline 12a was obtained, along with a small amount of meta -carbonyl phenol 2a , presumably because of a certain amount of water introduced by hygroscopic DMSO. As aforementioned, the reaction could also proceed with an excellent yield when tert -butyl hydroperoxide (TBHP) took the place of AgOAc and O 2 . After extensive screening of the reaction conditions (see Supplementary Tables 9 – 12 for optimization details), the desired meta -carbonyl aniline 12a was delivered in 73% yield in the presence of CuI (10 mol%), TBHP (2.2 equiv) and trifluoroacetic acid (TFA, 10.0 equiv) in DMSO (0.25 M) at 90 o C for 60 h. With optimal conditions in hand, we subsequently evaluated the scope of anilines 11 by using cyclohexyl(phenyl)methanone 1a as a model partner (Fig. 3a ). Anilines bearing electron-donating or electron-withdrawing groups were feasible, producing desired meta -carbonyl diphenylamines in 57–85% yield ( 12a - 12p ). Substituents at the otho , meta , or para positions were amenable to the catalytic system. Various functional groups, including Me, OMe, i Pr, t Bu, OPh, F, Cl, Br, and I, were also found to be suitable for this transformation. In addition, multi-substituted anilines also proved applicable under the standard conditions, furnishing the meta -carbonyl anilines in up to 89% yield ( 12q - 12w ). Gratifyingly, the 4-methoxyphenyl (PMP) group in 12m could be easily removed via the oxidation with cerium(IV) ammonium nitrate to deliver primary amine product (Supplementary Information Section 5.7 ). The structures of 12i and 12k were unambiguously confirmed by single-crystal X-ray diffraction (Supplementary Information Section 6 ). Fig. 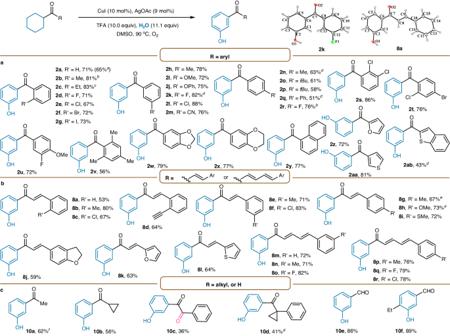Fig. 2: Substrate scope for synthesis ofmeta-carbonyl phenols. aSubstrate scope of aryl ketones.bSubstrate scope of conjugated enones.cSubstrate scope of aliphatic ketones and aldehydes. Reaction conditions: substrate (0.25 mmol), CuI (10 mol%), AgOAc (9 mol%), and TFA (10.0 equiv) in DMSO (1 mL), H2O (50 μL) under O2at 90oC for 60 h. Isolated yields are reported.aReaction conducted with 1a (5.5 mmol).bAgOAc (9.5 mol%) was used.c48 h.d100oC.eNo addition of H2O.fPd(OAc)2(15 mol%) was used instead of AgOAc. 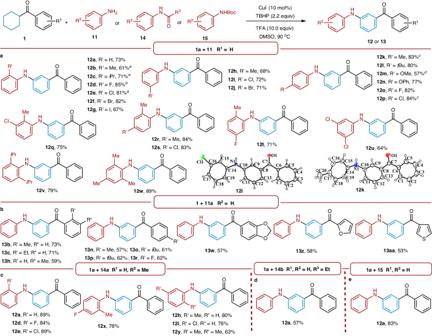Fig. 3: Substrate scope for synthesis ofmeta-carbonyl anilines. aSubstrate scope of anilines.bSubstrate scope of aromatic ketones.cSubstrate scope ofN-acetyl anilines.dSubstrate ofN-propionyl aniline.eSubstrate ofN-tert-butoxycarbonyl aniline. Reaction conditions:1(0.25 mmol),11(0.5 mmol) or14(0.5 mmol) or 15 (0.5 mmol), CuI (10 mol%), TBHP (2.2 equiv), and TFA (10.0 equiv) in DMSO (1 mL) at 90oC for 60 h. Isolated yields are reported.aTBHP (1.1 equiv).bTBHP (2.0 equiv).c36 h.dAgOAc (9 mol%) instead of TBHP. Boc,tert-butoxycarbonyl. 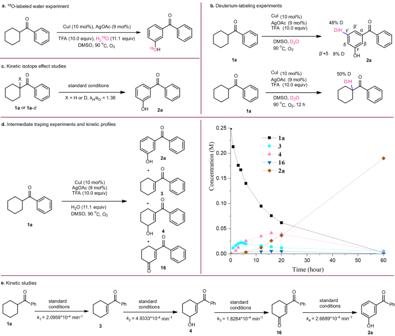Fig. 4: Mechanistic investigation. a18O-labeled water experiment.bDeuterium-labeling experiments.cKinetic isotope effect studies.dIntermediate traping experiments and kinetic profiles.eKinetic studies. 3: Substrate scope for synthesis of meta -carbonyl anilines. a Substrate scope of anilines. b Substrate scope of aromatic ketones. c Substrate scope of N -acetyl anilines. d Substrate of N -propionyl aniline. e Substrate of N - tert -butoxycarbonyl aniline. Reaction conditions: 1 (0.25 mmol), 11 (0.5 mmol) or 14 (0.5 mmol) or 15 (0.5 mmol), CuI (10 mol%), TBHP (2.2 equiv), and TFA (10.0 equiv) in DMSO (1 mL) at 90 o C for 60 h. Isolated yields are reported. a TBHP (1.1 equiv). b TBHP (2.0 equiv). c 36 h. d AgOAc (9 mol%) instead of TBHP. Boc, tert -butoxycarbonyl. Full size image We further surveyed the scope of aromatic ketones with aniline 11a (Fig. 3b ). Substrates bearing substituents with distinct electron properties on the aromatic ring moiety were feasible, delivering the corresponding products in moderate to good yields. Additionally, substituents at various positions were also viable for this strategy. Furthermore, heterocyclic substrates such as furyl and thienyl all occurred smoothly, also giving the expected products in 53–58% yield ( 13z and 13aa ). Encouraged by the foregoing success with anilines, we wondered whether the corresponding meta -carbonyl anilines could be obtained when using protected anilines instead of anilines. We then tested the reaction between protected anilines 14 and 15 and cyclohexyl(phenyl)methanone 1a (Fig. 3c–e ). Unexpectedly, protected anilines including N -acetyl aniline 14a, N -propionyl aniline 14b and N - tert -butoxycarbonyl aniline 15a all furnished the same deprotected product 12a in 89%, 57%, and 83% yields, respectively. N -acetyl anilines with electronically diverse substituents all proceeded smoothly, giving the meta -carbonyl deprotected anilines in good to excellent yields. In view of these results, we presumed that the protected anilines could be more stable than unprotected anilines under the oxidative conditions. Disubstituted substrates were also found to be compatible with the standard conditions, producing the desired products in good yields ( 12x and 12y ). Mechanistic investigation To gain insight into the reaction mechanism, a series of isotope tracking studies, deuterium-labeling experiments and kinetic studies were conducted. Initially, the 18 O-labeled water was introduced into the reaction system of 1a to probe the origin of the hydroxyl (Fig. 4a ). As a consequence, the 18 O-labeled product 2a was obtained by high-resolution mass spectrometry (HRMS) analysis, suggesting the hydroxyl in phenol did come from the water (Supplementary Fig. 5 ). Next, we carried out deuterium labeling experiments of 1a with D 2 O under the standard reaction conditions, providing the deuterium-labeling product with 48% D incorporation at the γ‘ position. In addition, the recovered 1a was found to contain 50% D at the α position (Fig. 4b ). The occurrence of H/D exchange indicates that this catalytic system enables the activation of the α -C−H and γ -C−H bond. Additionally, the kinetic isotope effect (KIE) experiments showed the value of k H / k D = 1.38 for parallel experiments of 1a and 1a - d , indicating that the cleavage of the α -C−H bond may not be involved in the rate-limiting step (Fig. 4c ). Subsequently, intermediate trapping experiments were conducted using substrate 1a to shed light onto the reaction mechanism (Fig. 4d ). In addition to the desired product 2a , compounds 3, 4 , and 16 were also observed and isolated. To gain deeper understanding into the reaction process, we conducted a kinetic time course analysis of the reaction using 1 HNMR. Monitoring the reaction process via periodic sampling revealed that α,β -unsaturated ketone 3 is initially formed, allylation product 4 subsequently formed, and 1,4-enedione 16 ultimately formed. Compounds 3, 4 and 16 are subsequently consumed as the product 2a is formed. These results provided evidence to support that 3, 4 and 16 are reaction intermediates to produce the product 2a . We reasoned that synthesis of meta -carbonyl phenols proceeds through the following cascade ( 1a → 3 → 4 → 16 → 2a ). To obtain kinetic rate constants of each step, the substrate 1a and intermediates 3, 4 and 16 were subjected to the standard conditions, respectively (Fig. 4e ). The rate constants for each step were determined as follows: k 1 = 2.0959 × 10 −4 min −1 , k 2 = 4.9333 × 10 −4 min −1 , k 3 = 1.8284 × 10 −4 min −1 , k 4 = 2.6889 × 10 −4 min −1 , giving a ratio of k 1 / k 2 / k 3 / k 4 = 1.15:2.70:1.00:1.47. These results indicated that the allylic oxidation of 4 to 16 was the rate-limiting step. Based on the experimental results and the related literature [37] , [38] , [39] , a plausible reaction mechanism for synthesis of meta -carbonyl phenols or anilines was proposed (Supplementary Fig. 23 ). Fig. 4: Mechanistic investigation. a 18 O-labeled water experiment. b Deuterium-labeling experiments. c Kinetic isotope effect studies. d Intermediate traping experiments and kinetic profiles. e Kinetic studies. Full size image In conclusion, we have established an efficient synthetic protocol for meta -substituted phenols and anilines. The approach is simple, proceeds under mild conditions, and uses abundant and inexpensive copper catalysts, rendering it practical advantages. Furthermore, this transformation is of complete meta -site selectivity, and no ortho - and/or para -isomers were detected, which facilitates subsequent purification processes. We anticipate that this strategy will be useful for the synthesis of other meta -functionalized aromatic compounds. General procedure for the synthesis of meta -carbonyl phenols A 15 mL sealed tube containing a magnetic stir bar was charged with ketones (0.25 mmol), CuI (4.8 mg, 10 mol%), AgOAc (3.7 mg, 9 mol%), and DMSO (1 mL) sequentially. The tube was evacuated and backfilled with O 2 three times. Subsequently, H 2 O (50 μL, 11.1 equiv) and TFA (186 μL, 10.0 equiv) were added. The tube was sealed and the mixture was stirred at 90 °C for 60 h. After cooling to room temperature, the reaction mixture was diluted with EtOAc (50 mL) and washed with H 2 O (3 × 1 mL) and brine (3 × 1 mL). The combined organic layer was dried over anhydrous Na 2 SO 4 , and concentrated to give the residue, which was further purified by silica gel column chromatography to afford the desired product. General procedure for the synthesis of meta -carbonyl anilines A 15 mL sealed tube containing a magnetic stir bar was charged with ketones (0.25 mmol), anilines (0.5 mmol), CuI (4.8 mg, 10 mol%), DMSO (1 mL) and TFA (186 μL, 10.0 equiv) sequentially. Subsequently, TBHP (100 μL, 2.2 equiv) was added. The tube was sealed and the mixture was stirred at 90 °C for 60 h. After cooling to room temperature, the reaction mixture was diluted with EtOAc (50 mL) and washed with H 2 O (3 × 1 mL) and brine (3 × 1 mL). The combined organic layer was dried over anhydrous Na 2 SO 4 , and concentrated to give the residue, which was further purified by silica gel column chromatography to afford the desired product.